Northern-hemispheric differential warming is the key to understanding the discrepancies in the projected Sahel rainfall Future projections of the Sahel rainfall are highly uncertain, with different climate models showing widely differing rainfall trends. Moreover, the twentieth-century cross-model consensus linking Sahel rainfall to tropical sea-surface temperatures (SSTs) is no longer applicable in the twenty-first century. Here we show that the diverse future Northern Hemisphere differential warming between extratropical and tropical SSTs can explain the discrepancy in the projected Sahel rainfall. The relationship between SST and Sahel rainfall that holds for the twentieth-century persists into the twenty-first century when the differential SST warming is taken into account. A suite of SST-sensitivity experiments confirms that strong Northern Hemisphere extratropical warming induces a significant increase in Sahel rainfall, which can predominate over the drying impact of tropical SST warming. These results indicate that a trustworthy projection of Sahel rainfall requires the estimation of the most likely future Northern-hemispheric differential warming. The semiarid Sahel, located south of the Sahara desert, has its rainy season in the boreal summer. The rainfall over the African Sahel region exhibits puzzling behaviour in twenty-first century projections [1] , [2] , [3] , [4] , [5] , [6] . Future Sahel rainfall projections in different climate models disagree, even on the direction of the trend. Given the robust drying in response to late twentieth-century forcing factors of the same coupled models [7] , such a disagreement with respect to future Sahel rainfall is surprising. Apart from the question of whether Sahel rainfall will increase or decrease, how such disparate Sahel rainfall projections arise remains an open question. Sea-surface temperature (SST) variations are recognized to be the main cause of the observed decadal Sahel rainfall variability [8] , [9] , [10] , [11] , [12] , with local soil moisture or vegetation feedbacks only amplifying the SST-driven low-frequency variability [13] . However, an attempt to predict future Sahel rainfall based on its historical relationship with tropical SSTs has been unsuccessful [1] . Alternative explanations have been proposed regarding the source of the model discrepancy, such as the strength of the Sahara Low and the land surface response to radiative forcing [14] , [15] . Given that oceanic forcing has played a dominant role in shaping the observed decadal variations of Sahel rainfall and previous studies mainly restricted their analysis to tropical SSTs to predict future rainfall changes, it is necessary to extend the investigation to the role of global SSTs to understand the disagreement in predicted Sahel rainfall trends. In this study, we show that SSTs are the fundamental factor in estimating future Sahel rainfall changes. The difference between future scenarios and the historical period is that the key SST area determining future Sahel rainfall changes will be shifted from the tropics to the Northern Hemisphere (NH) extratropics in the case of dominant future extratropical warming over tropical warming. A multi-model analysis reveals that future Sahel rainfall change can be substantially modified by the magnitude of extratropical warming, which is also confirmed by a series of SST-sensitivity experiments. A confident projection of future Sahel rainfall requires an understanding of the cause of the discrepancy in rainfall predictions in current climate models, and here, we contribute to such understanding by establishing NH differential warming as a crucial factor underlying the uncertainty regarding future Sahel rainfall. Statistical analysis of multi-model outputs in CMIP5 The uncertainty in future Sahel rainfall found in the third phase of the Coupled Model Intercomparison Project (CMIP3) models is present even in the new generation of climate models, that is, CMIP5 ( Fig. 1a and Supplementary Fig. 1 ). For example, as shown in the future projection from ‘gfdl-cm2.1’ and ‘miroc3_2_medres’ in CMIP3 (refs 1 , 2 ), two CMIP5 models from the same family, GFDL-ESM2M and MIROC-ESM, still project a substantially dryer and wetter Sahel, respectively, under a medium future emission scenario (Representative Concentration Pathways 4.5; RCP4.5). A recent study using the strongest radiatively forced future scenario for CMIP5 also supports the model variability of future Sahel rainfall trends [16] . We cannot ignore those two extreme simulations because either the drying or wetting of the Sahel is a physically plausible response to increased radiative forcing, and these two models provide relatively accurate simulations of the West African summer rainfall in the historical period [3] . 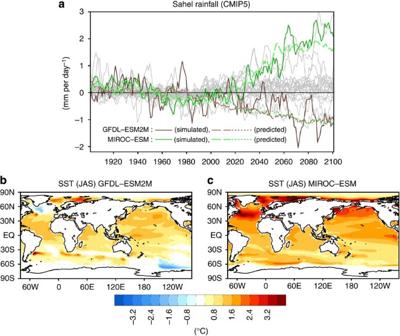Figure 1: Uncertainty in future Sahel rainfall and global SST warming pattern. (a) The JAS mean Sahel rainfall (10°W–30°E; 10°–20°N) anomalies during the twentieth and twenty-first centuries from CMIP5 models. Brown- and green-solid lines represent the Sahel rainfall anomalies simulated by GFDL-ESM2M and MIROC-ESM, which produce extreme Sahel drying and wetting, respectively. The rainfall anomalies from other CMIP5 models are indicated by grey lines. Dotted lines are the linearly predicted Sahel rainfall anomalies based on two tropical SST indices: the Atlantic SST gradient [(70°–20°W, 5°–30°N) minus (40°W–5°E, 30°S–5°N)] and Indo-Pacific SST (50°E–90°W, 20°S–20°N). Dashed lines represent predicted Sahel rainfall anomalies using an extratropical SST index (0°–360°E, 30°–75°N) in addition to the two tropical indices. The regression coefficients of the multi-linear model are calculated from the historical simulation (1901–2005). The anomalies are the differences from the historical mean and all time series data are smoothed using a 5-year running mean. (b,c) JAS SST differences between the twenty-first century and twentieth-century for GFDL-ESM2M (b) and for MIROC-ESM (c). Figure 1: Uncertainty in future Sahel rainfall and global SST warming pattern. ( a ) The JAS mean Sahel rainfall (10°W–30°E; 10°–20°N) anomalies during the twentieth and twenty-first centuries from CMIP5 models. Brown- and green-solid lines represent the Sahel rainfall anomalies simulated by GFDL-ESM2M and MIROC-ESM, which produce extreme Sahel drying and wetting, respectively. The rainfall anomalies from other CMIP5 models are indicated by grey lines. Dotted lines are the linearly predicted Sahel rainfall anomalies based on two tropical SST indices: the Atlantic SST gradient [(70°–20°W, 5°–30°N) minus (40°W–5°E, 30°S–5°N)] and Indo-Pacific SST (50°E–90°W, 20°S–20°N). Dashed lines represent predicted Sahel rainfall anomalies using an extratropical SST index (0°–360°E, 30°–75°N) in addition to the two tropical indices. The regression coefficients of the multi-linear model are calculated from the historical simulation (1901–2005). The anomalies are the differences from the historical mean and all time series data are smoothed using a 5-year running mean. ( b , c ) JAS SST differences between the twenty-first century and twentieth-century for GFDL-ESM2M ( b ) and for MIROC-ESM ( c ). Full size image In addition to the opposing Sahel rainfall projections, the two models show a substantial difference in their projections of future Northern-hemispheric SST warming ( Fig. 1b,c ). In GFDL-ESM2M, the amplitudes of tropical and extratropical SST warming are similar, whereas in MIROC-ESM, extratropical warming is more prominent than warming in the tropics, particularly in the NH. Such association between strong NH extratropical SST warming and Sahel wetting or between weak warming and Sahel drying over the next century can also be found in other models ( Supplementary Fig. 2 ). Therefore, we will investigate the role of NH extratropical SST warming in forcing the contradictory projections of future Sahel rainfall. The MIROC models are key to understanding the discrepancy in the future projections because of a strong positive trend of future Sahel rainfall and a strong extratropical SST warming. Thus, the role of NH extratropical SST in predicting future Sahel rainfall is evaluated by reconstructing the simulated rainfall from MIROC-ESM based on different combinations of SST indices. First, the Sahel rainfall is linearly reconstructed using only commonly used tropical indices, namely, the interhemispheric SST gradient index in the tropical Atlantic ((70°–20°W, 5°–30°N) minus (40°W–5°E, 30°S–5°N)) and the area-averaged Indo-Pacific SST index (50°E–90°W, 20°S–20°N). The statistical model and indices are similar to those used in previous studies [1] , [5] . The two tropical indices reconstruct the Sahel rainfall reasonably well in the historical run, whereas they fail to reconstruct the future Sahel rainfall, exhibiting a drying trend in future Sahel rainfall (dotted green line in Fig. 1a ). This shortcoming confirms that the previously used tropical SST indices are insufficient to predict a strong positive trend of future Sahel rainfall. In contrast, inclusion of the extratropical SST index (0°–360°E, 40°–75°N) in the statistical model reconstructs future Sahel rainfall considerably well with the strong positive trend similar to the simulated Sahel rainfall (dashed green line in Fig. 1a ). Using a single index of NH differential SST warming ((0°–360°E, 30°–75°N) minus (0°–360°E, 20°S–20°N)) in the statistical model also successfully reproduces the strong positive trend ( Supplementary Fig. 3a ). Such an improved reproduction of future Sahel rainfall when considering the extratropical SST warming is not found in a similar analysis with a drying model (that is, GFDL-ESM2M, dashed brown line almost overlapped by the dotted brown line in Fig. 1a ), a result that could be expected from the weak future NH extratropical warming simulated by GFDL-ESM2M. Notably, the future development of Sahel rainfall can be reconstructed simply based on twentieth century relationships with large-scale SST indices including NH extratropical SST. That is, during the historical period Sahel rainfall is mainly affected by tropical SSTs because the extratropical SST plays a minor role due to the weak magnitude of its anomalies. However, if the NH extratropical SST warming becomes stronger under a global warming scenario compared with the warming in the tropics, then the future Sahel rainfall changes cannot be explained solely by tropical SST changes. Rather, the extratropical SST should be taken into account. We further investigate how much the future Sahel rainfall change is related to the NH differential warming across the CMIP5 models. Future changes in Sahel rainfall and those in the NH differential warming are calculated in each CMIP5 model and displayed in a scatter plot ( Fig. 2a ). Models showing a stronger extratropical warming relative to the tropics tend to project a wetter Sahel. The relationship is quite robust despite other possible factors influencing future Sahel rainfall changes (for example, local land-surface or land-atmosphere feedbacks, intermodel variations in future tropical SST anomalies and different model sensitivities to SST forcing). On the basis of the fitted linear line, the same magnitude of warming over extratropical and tropical oceans leads to drying conditions over the Sahel, which is consistent with a drying Sahel rainfall response to globally uniform warming shown in a previous work [11] . 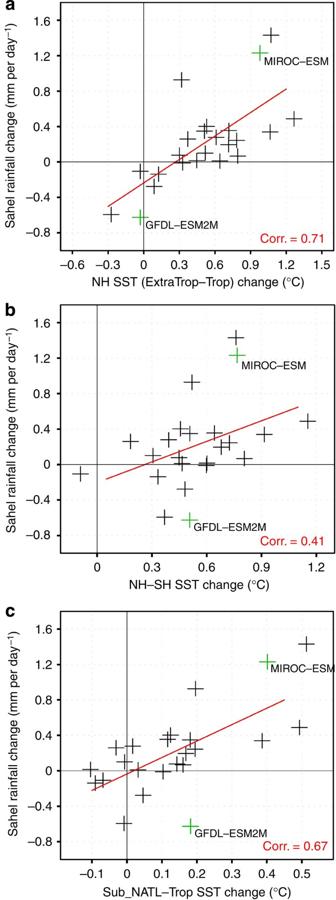Figure 2: Performance of various SST indices in explaining future Sahel rainfall change. (a–c) Scatter plots of future changes (that is, mean difference between the twenty-first century and twentieth-century) in Sahel rainfall versus those in three different SST indices across the CMIP5 models: NH extratropical SST warming relative to tropical warming ((0°–360°E, 30°–75°N) minus (0°–360°E, 20°S–20°N)) (a), global interhemispheric SST gradient ((0°–360°E, 0°–90°N) minus (0°–360°E, 0°–90°S)) (b) and difference between subtropical North Atlantic SST and global tropical SST ((75°–15°W, 10°–40°N) minus (0°–360°E, 20°S–20°N)) (c). Each mark represents an individual model in CMIP5. The fitted linear regression lines are shown as red lines. Figure 2: Performance of various SST indices in explaining future Sahel rainfall change. ( a – c ) Scatter plots of future changes (that is, mean difference between the twenty-first century and twentieth-century) in Sahel rainfall versus those in three different SST indices across the CMIP5 models: NH extratropical SST warming relative to tropical warming ((0°–360°E, 30°–75°N) minus (0°–360°E, 20°S–20°N)) ( a ), global interhemispheric SST gradient ((0°–360°E, 0°–90°N) minus (0°–360°E, 0°–90°S)) ( b ) and difference between subtropical North Atlantic SST and global tropical SST ((75°–15°W, 10°–40°N) minus (0°–360°E, 20°S–20°N)) ( c ). Each mark represents an individual model in CMIP5. The fitted linear regression lines are shown as red lines. Full size image A similar statistical analysis is conducted with alternative choices of previously known indices, which also include possible extratropical factors associated with Sahel rainfall, such as the global interhemispheric SST gradient [17] or the SST difference between the subtropical North Atlantic and the global tropical oceans [18] . We found that none of these indices performs comparably well to the NH intrahemispheric SST warming index ( Fig. 2b,c and Supplementary Fig. 3b,c ). For example, the regression model with these supplementary indices predicts a much weaker positive future rainfall trend than that with our NH differential warming SST index (see Supplementary Fig. 3a and Fig. 3b,c ). The more successful reproduction of Sahel rainfall when using our NH differential warming index also holds for the historical period ( Supplementary Fig. 4 and Supplementary Note 1 ). In addition, the two supplementary SST indices are less successful in consistently explaining future Sahel rainfall changes across the CMIP5 models (see Fig. 2a–c ). Although the SST index of subtropical North Atlantic minus global tropics shows a comparable correlation with future Sahel rainfall changes, it has some limitations. For example, the relative subtropical index cannot explain the opposite future rainfall anomalies in GFDL-ESM2M and MIROC-ESM, which are key models for diverse future projections. In addition, the subtropical index shows nearly zero rainfall change corresponding to uniform global warming, which is not consistent with previous work showing a drying Sahel in response to globally uniform warming [11] . Taken together, these results highlight the distinct role of NH differential warming for future Sahel rainfall, and the model discrepancy in future Sahel rainfall projections appears to arise from different magnitudes of NH extratropical warming simulated by CMIP5 models. 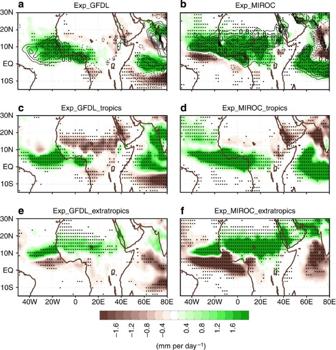Figure 3: Precipitation responses to SST sensitivity experiments. (a–f) Mean differences in summer (JAS) precipitation between the two experiments: the ‘21C run’ forced by twenty-first century (2070–2099) climatological SST and the ‘20C run’ forced by twentieth century (1970–1999) climatological SST from GFDL-ESM2M (a) and MIROC-ESM (b) in CMIP5. (c,d) are the same as (a,b) but for prescribing the twentieth century extratropical SST and the twenty-first century tropical SST for the ‘21C run’. Similarly,e,fare precipitation responses when considering the extratropical SST warming only. Contours ina,brepresent the superposition of the precipitation responses from tropical and extratropical SST experiments. The stippled area denotes the 95% confidence region according to two-tailedt-test. Figure 3: Precipitation responses to SST sensitivity experiments. ( a – f ) Mean differences in summer (JAS) precipitation between the two experiments: the ‘21C run’ forced by twenty-first century (2070–2099) climatological SST and the ‘20C run’ forced by twentieth century (1970–1999) climatological SST from GFDL-ESM2M ( a ) and MIROC-ESM ( b ) in CMIP5. ( c , d ) are the same as ( a , b ) but for prescribing the twentieth century extratropical SST and the twenty-first century tropical SST for the ‘21C run’. Similarly, e,f are precipitation responses when considering the extratropical SST warming only. Contours in a , b represent the superposition of the precipitation responses from tropical and extratropical SST experiments. The stippled area denotes the 95% confidence region according to two-tailed t -test. Full size image AGCM experiments forced by future SST warming Although the statistical analyses clearly emphasize the role of Northern-hemispheric differential heating as a possible source of diverse future projections of Sahel rainfall, we must verify whether the statistical link is physically consistent. Thus, a series of SST-sensitivity experiments with an atmospheric general circulation model (AGCM) has been conducted to yield more robust results and to understand the underlying processes. The model used here is the ECHAM6 (ref. 19 ), the atmospheric component of MPI-ESM-LR that shows nearly neutral conditions for the future Sahel rainfall under the RCP4.5 scenario ( Supplementary Fig. 1 ). The ECHAM6 is forced by the monthly climatological SSTs (averaged over the last 30 years of the twentieth and twenty-first centuries) from both GFDL-ESM2M and MIROC-ESM models in CMIP5. Hence, the difference in precipitation responses between the experiments prescribing twentieth and twenty-first century SSTs represents the impact of future global SST warming on Sahel rainfall. The ECHAM6 experiments forced by the global SST warming from GFDL-ESM2M and MIROC-ESM show a significant difference in Sahel rainfall, with a weak Sahel drying in the experiment using GFDL SST and a strong wetting in the MIROC SST case ( Fig. 3a,b ). Thus, the AGCM experiment is qualitatively consistent with the drying and wetting Sahel as simulated by GFDL-ESM2M and MIROC-ESM, respectively, in CMIP5. Note that the rainfall responses from our AGCM experiments can be further amplified if the interactive land and vegetation feedbacks, which are known to increase SST-driven Sahel rainfall changes [13] , are included in the experiments. This effect highlights the importance of the projected SSTs for the future development of Sahel rainfall and shows that the difference in the projected SSTs can largely explain the divergence of future Sahel rainfall projections. Furthermore, as noted above, the AGCM used for our experiments belongs to one of the CMIP5 models showing neutral conditions for the future Sahel rainfall. This condition leads us to hypothesize that different NH future SST anomalies may be a more dominant source of uncertainty in Sahel rainfall projections than different model sensitivities to the same SST forcing, although further experiments performed with a different AGCM are required to test this hypothesis. The individual impact of extratropical and tropical SST warming on Sahel rainfall was also evaluated by forcing ECHAM6 with the future SST warming restricted to the tropical and extratropical SST parts separately. The interesting finding here is that tropical SST warming induces less precipitation over the Sahel regardless of whether GFDL or MIROC SSTs are used ( Fig. 3c,d ). The difference in the magnitude of Sahel drying is presumably due to the varying patterns and magnitudes of tropical SST anomalies simulated by the two coupled models. For example, the stronger subtropical Atlantic warming in MIROC-ESM than in GFDL-ESM2M may induce less drying over the Sahel by increasing the moisture flux from the Atlantic Ocean. In contrast, both GFDL and MIROC SSTs produce an increase in Sahel rainfall when driven by the extratropical SST warming only ( Fig. 3e,f ). In particular, there is a strong wetting over the Sahel when the SSTs from MIROC-ESM are used, which confirms the conclusions of our previous statistical analysis using CMIP5 data. This result suggests that the precipitation decrease in GFDL-ESM2M, which shows less warming in the extratropics, is more affected by tropical warming, whereas the strong precipitation increase in MIROC-ESM is more influenced by strong extratropical warming. In other words, whether a model projects strong wet conditions over the Sahel depends on the dominance of extratropical warming over tropical warming. Because we argue that the future Sahel rainfall change can be explained by the competition between the two opposing impacts of tropical and extratropical warming, the linearity of the model response is tested. The superposition of two precipitation responses from the tropical and extratropical experiments shows a remarkable similarity to the precipitation response from the global SST warming experiment, which supports the conclusion that the precipitation response to global SST warming in our model experiments can be satisfactorily obtained by the linear combination of precipitation responses to tropical and extratropical SST warming ( Fig. 3a,b ). We also examined the direct radiative impact of CO 2 increase (not mediated by SST change) on Sahel rainfall. Additional AGCM experiments forced by increased CO 2 concentrations with fixed twentieth century mean SSTs show that the Sahel rainfall slightly increases independently of the GFDL or MIROC SSTs. This result indicates that the direct radiative CO 2 impact cannot be a source of the variability in predictions of future Sahel rainfall ( Supplementary Fig. 5 and Supplementary Note 2 ). Mechanisms of Sahel wetting by NH differential heating Because of the dominant role of tropical oceans on Sahel rainfall during the historical period [1] , [6] , several mechanisms proposed by previous studies can be applied to explain the relationship between warming tropical oceans and drying Sahel. Such mechanisms include the reduced ascent at certain convective margins due to the higher moisture requirement for convective instability (the so-called ‘upped-ante mechanism’) [20] , [21] , anomalous subsidence over the Sahel caused by tropical ocean warming [8] , [22] , [23] and weakened monsoonal flow due to the weaker contrast between ocean and continental temperatures [10] . In contrast, the role of extratropical SST warming on the Sahel rainfall has been relatively less studied. One might argue that the global interhemispheric SST gradient pattern shown in Fig. 1c is an extratropical factor inducing the Sahel rainfall increase by shifting the tropical rain belt to the north [24] , [25] (see also Fig. 2b and Supplementary Fig 3b ). However, the zonal mean precipitation change in the extratropical warming experiment clearly indicates that the Sahel rainfall increase is only partially explained by a northward rain belt shift, and more important factors associated with the Sahel rainfall intensity change are involved given the meridionally asymmetric rainfall anomalies ( Supplementary Fig. 6 ). Thus, we suggest potential mechanisms for how the NH differential warming is linked to the increase in Sahel rainfall by further analysing the strong extratropical warming experiment (Exp_MIROC_extratropics). One factor is the increased moisture flux driven by anomalous subtropical low pressure over North Africa and adjacent oceans ( Fig. 4a ). The large-scale low-pressure anomaly can deepen the Sahara Low, a main driver of the West Africa monsoonal wind, and thus intensify the westerly flow over the tropical Atlantic Ocean and West Africa. Consequently, the anomalous westerly moisture flux enhances moisture convergence over the Sahel, and in turn increases the rainfall. Given this connection between the NH extratropical warming and Sahel rainfall increase, our results are consistent with previous works. For example, one study showed that the increased temperature and atmospheric humidity advected from the extratropics can induce a positive long-wave radiation moisture feedback and either maintain or further amplify the surface warming over North Africa [26] . This finding provides a favourable condition for the Sahel rainfall increase due to the strengthening of the land-sea thermal contrast (associated with a strong monsoon flow) and the increased moist static energy (associated with a northward shift of the climatological rain belt) [26] , [27] . Another study suggested the role of the Sahara Low as a possible source of the variation in future Sahel rainfall projections [14] . The disparate magnitudes of NH differential warming emphasized in the present study may be an underlying cause of the different Sahara Low intensities projected by climate models, leading to the diverse projections of Sahel rainfall. 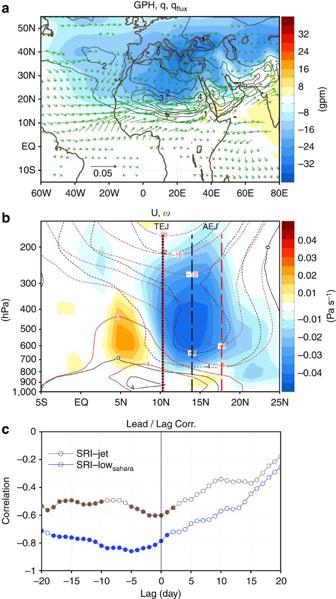Figure 4: Mechanisms for associating NH differential heating with Sahel rainfall increase. (a) The JAS mean difference in 925-hPa geopotential height (shadings, unit: m), moisture (contours, unit: 10−3kgH2Okgair−1) and moisture flux (arrows, unit:kgH2Okgair−1m s−1) between the two experiments, MIROC_21C_extratropics and MIROC_20C. The difference in moisture flux is only plotted where the mean difference is statistically significant, exceeding the 95% confidence level according to a two-tailedt-test. (b) Zonally averaged (10°W–30°E) zonal wind from MIROC_20C (black contours) and MIROC_21C_extratropics (red contours). Vertical lines represent axes of TEJ (dotted lines) and AEJ (dashed lines) for MIROC_20C (black) and for MIROC_21C_extratropics (red). Shading represents the JAS mean difference between MIROC_21C_extratropics and MIROC_20C. (c) Lead/Lag correlations between Sahel rainfall (10°W–30°E; 10°–20°N) and Sahara Low (10°W–30°E; 20°–30°N) and between Sahel rainfall and upper-level tropical easterly jet (10°W–30°E; 5°–15°N). The ensemble-mean daily data are used for this analysis. Negative lag indicates that Sahara Low and jets lead the Sahel rainfall. Filled circles represent correlations exceeding the 90% confidence level. Figure 4: Mechanisms for associating NH differential heating with Sahel rainfall increase. ( a ) The JAS mean difference in 925-hPa geopotential height (shadings, unit: m), moisture (contours, unit: 10 −3 kg H 2 O kg air − 1 ) and moisture flux (arrows, unit: kg H 2 O kg air − 1 m s −1 ) between the two experiments, MIROC_21C_extratropics and MIROC_20C. The difference in moisture flux is only plotted where the mean difference is statistically significant, exceeding the 95% confidence level according to a two-tailed t -test. ( b ) Zonally averaged (10°W–30°E) zonal wind from MIROC_20C (black contours) and MIROC_21C_extratropics (red contours). Vertical lines represent axes of TEJ (dotted lines) and AEJ (dashed lines) for MIROC_20C (black) and for MIROC_21C_extratropics (red). Shading represents the JAS mean difference between MIROC_21C_extratropics and MIROC_20C. ( c ) Lead/Lag correlations between Sahel rainfall (10°W–30°E; 10°–20°N) and Sahara Low (10°W–30°E; 20°–30°N) and between Sahel rainfall and upper-level tropical easterly jet (10°W–30°E; 5°–15°N). The ensemble-mean daily data are used for this analysis. Negative lag indicates that Sahara Low and jets lead the Sahel rainfall. Filled circles represent correlations exceeding the 90% confidence level. Full size image Another possible link between the NH differential warming and the increase in Sahel rainfall can be found in upper-level jets over Africa. Two tropical jets, the Tropical Easterly Jet (TEJ) and the African Easterly Jet (AEJ), are upper-level circulation factors known to influence Sahel rainfall [28] . The intensity of the TEJ, which modulates the divergence and uplift in the upper troposphere, is associated with rainfall anomalies over much of western Africa [29] , [30] , [31] , and the location of the AEJ is linked to the latitudinal extent of the atmospheric ascent and the tropical rain belt over West Africa [28] , [29] . We found that the responses of these two jets in our extratropical warming experiment are in agreement with the observed relationship between the jets and Sahel rainfall. The TEJ is significantly intensified in the presence of extratropical warming, whereas the AEJ shifts northward by ~4° over the Sahel region with relatively little change in its magnitude ( Fig. 4b ). Such circulation features are consistent with the anomalous ascending motion over the Sahel and the corresponding rainfall increase ( Fig. 4b , and Supplementary Fig. 6 ). Although the aforementioned explanation is physically plausible and is consistent with previous observational results, it does not provide clear evidence of causal relationships. For example, changes in the Sahara Low or the upper-level jet might be caused by the increased precipitation. To clarify this uncertainty, both the lead–lag relationships between Sahel rainfall and the strength of Sahara Low, and between Sahel rainfall and the intensity of TEJ were analysed by using daily model outputs ( Fig. 4c ). We found that the changes both in the Sahara Low and jet strength generally precede Sahel rainfall change. Therefore, the change in atmospheric dynamics is likely to be a cause, rather than a consequence, of the substantial increase in Sahel rainfall. Similar to the atmospheric response over North Africa to the NH extratropical warming, tropical Atlantic SST warming can also result in an increase in Sahel rainfall with the intensification of the Sahara heat low and the increased low-level moisture flux [32] , [33] . However, the moistening impact of the specific warming pattern in the tropics is relatively weak in a warming climate, thus the drying impact by the warming of the Indian and Pacific oceans dominates the Sahel rainfall response as shown in our tropical SST experiments. Specifically, if the future extratropical warming is stronger than the tropical warming, the extratropical impact on the Sahara Low or Sahel rainfall is expected to dominate subtropical/tropical impacts. A previous modelling work based on the historical period also supports this relation, showing that tropical Atlantic warming alone cannot fully explain Sahel rainfall responses to North Atlantic warming (see Figs 3j,k and 4j,k in Sutton and Hodson [33] ). The proposed connections linking strong future extratropical warming and Sahel rainfall increase may be relevant to previous findings, particularly focused on the extratropical North Atlantic Ocean. For example, the extratropical North Atlantic cooling associated with Atlantic multi-decadal variability is known to reduce Sahel rainfall by the advection of cold, dry air to North Africa and corresponding changes in sea-level pressure and moist static energy [26] . The mid-tropospheric Rossby-wave activity originated from the North Atlantic is also a possible atmospheric factor in linking extratropical energy to the African subtropical climate [34] . An additional AGCM experiment, however, shows that only approximately one-third of the total precipitation increase shown in Fig. 3f can be explained by extratropical Atlantic warming alone, indicating that SST warming in other ocean basins, such as the Mediterranean Sea and North Pacific and Arctic Oceans, also contributes substantially to the NH extratropical warming impact on Sahel rainfall. Over the past decade, the future projection of Sahel rainfall and the source of the discrepancies among the coupled GCMs has been an issue of great concern because of the historical climate-related calamities in this vulnerable area. Our results demonstrate that the NH differential warming is the crucial factor in consistently explaining the previously reported conundrum of future Sahel rainfall behaviour. In contrast to the observed period in which Sahel rainfall change is mainly driven by tropical SSTs, the moistening impact of strong extratropical SST warming is expected to dominate over the drying impact of tropical SST warming for the future Sahel rainfall, suggesting a fundamental shift in the pathway of SST impact in a warming climate. Therefore, a careful investigation of how the NH SST responds to greenhouse gas-induced warming is of great importance to obtain more reliable estimates of future Sahel rainfall. Given a relatively long predictability of extratropical SST [35] , a better understanding and determination of the factors controlling extratropical surface warming is likely the critical issue for improving the reliability of decadal predictions and future projections of Sahel rainfall. CMIP5 archive The data analysed here are obtained from the CMIP5 multi-model outputs [36] . A total of 23 CMIP5 models, which provide SST and precipitation outputs during the period 1860–2100, are used in this study, focusing on the seasonal mean (July–September, JAS) values. In particular, much attention is devoted to analysing two models, ‘GFDL-ESM2M’ and ‘MIROC-ESM’, which project two opposite extreme anomalies of future Sahel rainfall. These two models originate from ‘gfdl_cm2_1’ and ‘miroc3_2_medres’ in CMIP3, which also predicted extreme drying and wetting, respectively. The two versions of models developed from the same modelling group are basically the same except for incorporating carbon dynamics and some minor tuning in physical models [37] , [38] . The future scenario chosen for the present study is the Representative Concentration Pathways 4.5 (RCP4.5), a mid-range mitigation scenario. All CMIP5 models used here are depicted in Supplementary Fig. 1 . Linear regression model to predict future Sahel rainfall The statistical model used in our study is equivalent to the conventional multi-linear regression method, which is a standard technique to estimate the predictand from two or more explanatory variables. The best-fit line is calculated by the least-squares method, minimizing the sum of the squares of the deviations from the fitted line. We used the regression coefficients from the historical run for the future Sahel rainfall prediction. A cross-validation test, which is performed by calculating the coefficients from the future period and applying them to predict the historical rainfall, confirms the robustness of the statistical model. Model and experimental design The ECHAM6 model, developed at the Max Planck Institute for Meteorology, is used for the SST sensitivity experiments. The ECHAM models are known to reproduce the African monsoon reasonably well and have been extensively used for West African monsoon studies [39] , [40] , [41] . The model is run at T63 horizontal resolution (1.875° × 1.875°) with 47 vertical levels. The SST fields prescribed in the model are obtained from two CMIP5 models: GFDL-ESM2M and MIROC-ESM. Note that the corresponding sea ice fields are also used for physical consistency. Each experiment basically consists of a pair of two experiments, named ‘20C run’ and ‘21C run’. In the 20C run, the model is forced by the monthly climatological mean SSTs over the last thirty years of the twentieth century (1970–1999), whereas in the 21C run the model is forced by those over the last 30 years of the twenty-first century (2070–2099). The precipitation anomalies shown in the present study represent the difference between these two experiments. In the case of isolating the impact of tropical SST, the prescribed SST in the extratropics (poleward of 30°) is fixed to the twentieth century SST (as in case in the 20C run) and only the tropical SST (30°S–30°N) from the twenty-first century is used for the 21C run (and vice versa for the case of extratropical SST). All other boundary conditions (for example, greenhouse gases and solar radiation) are identical for all integrations. A total of 20 ensemble members with different initial conditions are conducted, and only the JAS mean is shown in this study. A summary of the experimental design is provided in Supplementary Table 1 . How to cite this article: Park, J.-Y. et al . Northern-hemispheric differential warming is the key to understanding the discrepancies in the projected Sahel rainfall. Nat. Commun. 6:5985 doi: 10.1038/ncomms6985 (2015).